Tumour-derived SPARC drives vascular permeability and extravasation through endothelial VCAM1 signalling to promote metastasis Disruption of the endothelial barrier by tumour-derived secreted factors is a critical step in cancer cell extravasation and metastasis. Here, by comparative proteomic analysis of melanoma secretomes, we identify the matricellular protein SPARC as a novel tumour-derived vascular permeability factor. SPARC deficiency abrogates tumour-initiated permeability of lung capillaries and prevents extravasation, whereas SPARC overexpression enhances vascular leakiness, extravasation and lung metastasis. SPARC-induced paracellular permeability is dependent on the endothelial VCAM1 receptor and p38 MAPK signalling. Blocking VCAM1 impedes melanoma-induced endothelial permeability and extravasation. The clinical relevance of our findings is highlighted by high levels of SPARC detected in tumour from human pulmonary melanoma lesions. Our study establishes tumour-produced SPARC and VCAM1 as regulators of cancer extravasation, revealing a novel targetable interaction for prevention of metastasis. Metastasis is a challenging clinical problem and the primary cause of death from cancer. Tumour progression towards metastasis occurs by a complex multi-step process whereby tumour cells dissociate from their primary site of growth, invade surrounding tissues, intravasate into a blood vessel, survive in circulation, adhere to and extravasate from the vessel and form a new tumour at secondary site. The metastatic behaviour of cancer cells relies on both cell-autonomous and non-autonomous processes, the latter involving dynamic interactions with non-malignant cells within the tumour microenvironment [1] , [2] , [3] . Cutaneous melanoma is notorious for its proclivity for early and extensive metastatic spread and recognized as one of the most virulent and resistant to therapy of human cancers. In most cases, melanoma derives from an epidermal melanocyte and progresses into a primary tumour that can invade into the dermis and draining lymph nodes and from there disseminate to distant organs [4] , [5] . Early-stage melanomas can be successfully treated by surgical resection. However, patients with more advanced forms of melanomas have a much lower chance of long-term survival. Recent progresses in melanoma treatments have led to improved survival in patients with metastatic disease [6] , [7] . However, the prognosis remains still very poor for most patients. Thus, studies aiming at defining the driver mechanisms of metastatic dissemination could lead to novel therapeutic strategies that could improve clinical outcomes for melanoma patients. The mechanisms that mediate haematogenous metastatic formation depend, in part, on the ability of circulating tumour cells to exit the bloodstream through the blood vessel wall composed of endothelial cells, the basement membrane and perivascular cells, and enter the tissue parenchyma. The opening of endothelial junctions is the prelude for the transmigration process in which tumour cells can move through the junctions between adjacent endothelial cells thereby enabling metastatic seeding in the invaded organs [8] . This process is related to the well-studied physiological process of paracellular diapedesis of leukocytes during inflammation and requires disruption of the barrier function of the endothelium [9] . The paracellular permeability of the endothelium is regulated by the dynamic opening and closure of intercellular junctions. Transmembrane adhesion proteins are located at both adherens and tight junctions and function to connect adjacent endothelial cells and to sustain the barrier integrity [10] . The stability of these contacts is maintained by coordinated mechanisms on the basis of contractile forces produced by the acto–myosin complex and interaction of the actin cytoskeleton with adherens or tight junctions-associated proteins including β-catenin, α-catenin, zona occludens 1 (ZO1) and 2 (ZO2), and others [10] , [11] . The vascular endothelial cadherin (VE-cadherin) represents one of the major adhesion systems that support the endothelial barrier function. Signalling pathways that increase vascular permeability generally affect adhesive function of VE-cadherin, in part, through tyrosine phosphorylation of constituents of adherens junctions and activation of acto–myosin contractibility accompanied by reorganization of the actin cytoskeleton that cause formation of stress fibrer and intercellular gaps [8] , [12] . Vascular permeability is thus a complex phenomenon involving coordinated regulation of diverse signalling pathways in the endothelial cell. Within the malignant melanoma microenvironment, communication between tumour cells, their secreted factors and the endothelium is thought to increase paracellular vascular permeability. Thus, disruption of endothelium integrity by tumour cells appears as a critical and early event that facilitates extravasation, yet the way by which metastatic melanoma cells affect vascular permeability is not fully understood. Here, we have investigated the secreted factors and paracrine signalling pathways responsible for tumour-initiated vascular permeability during cancer cell extravasation in the context of melanoma metastasis. We identify the matricellular SPARC protein, as a critical tumour-secreted permeability factor and a novel paracrine mediator of endothelium permeability during melanoma metastatic dissemination to lungs. Abnormal expression of SPARC has been reported in various cancer cell types including melanoma [13] , in which SPARC was shown to play a key role in melanoma cell tumorigenicity [14] , [15] , [16] . However, its role as a paracrine mediator of haematogenous metastasis during extravasation remains unclear. We report here the first evidence that tumour cell-derived SPARC instigates the disruption of the endothelial barrier through binding to vascular cell adhesion molecule 1 (VCAM1) and activation of p38 MAPK-mediated signalling pathways leading to actin cytoskeleton re-organization and opening of endothelial intercellular junctions. Our study brings new and important insights into the mechanisms of tumour cell extravasation at the endothelial barrier during melanoma metastasis. Metastatic melanoma releases vascular permeability factors We reasoned that malignant melanoma cells produce secreted permeability factors and use paracrine signalling to communicate with the endothelial barrier to extravasate during metastatic dissemination. To address this issue, we prepared conditioned medium (CM) from normal human melanocytes (NHM) and a panel of melanoma cells displaying different metastatic potential ( Fig. 1a ) to analyse how these CM modulate endothelial permeability. Endothelial cell monolayer permeability has been evaluated in vitro using a FITC-Dextran Transwell assay ( Supplementary Fig. 1a ). Primary Human umbilical vein endothelial cells (HUVECs) grown to confluence were exposed to normal growth medium or to CM prepared from NHM or melanoma cell lines (1205Lu, A375, SKMel28 and 501Mel). The 501Mel cells were chosen because compared with the other melanoma cells used they show no metastatic potential in mice. We also analysed the effect of CM derived from short-term cultures of metastatic melanoma cells (Pt1, Pt2 and Pt3). As shown in Supplementary Fig. 1a , monolayer permeability was significantly higher following exposure to CM collected from 1205Lu, A375 and SKMel28 cell lines or from short-term cultures compared with CM collected from NHM. In contrast, CM derived from non-metastatic 501Mel cells did not greatly increase endothelial permeability when compared with the effect of CM prepared from the other melanoma cells. These results indicate that metastatic melanoma cell-derived CM contains factors that are sufficient to promote junctional permeability. 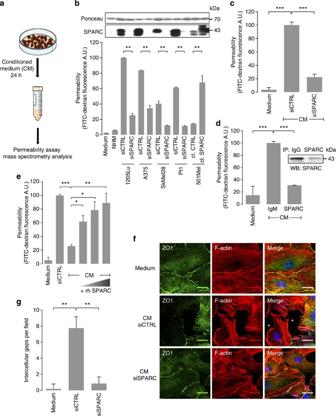Figure 1: Tumour-secreted SPARC reduces endothelial monolayer integrity. (a) Schematic representation of CM production from melanoma cell cultures. After 24 h, CM was collected and used for permeability assays or mass spectrometry analysis (seeSupplementary Fig. 1andSupplementary Data 1). (b) Primary endothelial cells (HUVECs) were seeded into gelatin-coated Boyden chambers, allowed to grow to confluence and then treated with TNFα (10 ng ml−1) overnight. Permeability was determined by a FITC-Dextran assay 7 h after addition of CM from melanoma cells depleted or not for SPARC by siRNA or from 501Mel cells stably overexpressing SPARC (cl. SPARC) or not (cl. CTRL). Bar graphs show mean±s.e.m.,n=2 independent experiments performed in triplicate. Upper panels show representative anti-SPARC blots. Ponceau staining was used as loading control. siCTRL, control siRNA; siSPARC, SPARC siRNA. (c) Permeability analysis of human pulmonary microvascular endothelial cells (HPMECs) 7 h after addition of 1205Lu CM depleted or not for SPARC. Bar graphs show mean±s.e.m.,n=2 independent experiments performed in triplicate. (d) Permeability of HUVECs was assayed using 1205Lu CM cleared from SPARC by immunoprecipitation (IP). Inset shows representative SPARC immunoblot analysis of the cleared CM. Bar graphs show mean±s.e.m.,n=2 independent experiments performed in triplicate. (e) Permeability assay was performed using CM from 1205Lu cell cultures depleted for SPARC by siRNA and rescued by recombinant human SPARC (rhSPARC). Increasing doses of rhSPARC were added in the upper chamber (2, 5 or 10 μg ml−1) and FITC-Dextran fluorescence was determined in the lower chamber 7 h after the addition of CM. Bar graphs show mean±s.e.m.,n≥3independent experiments performed in triplicate. (f) Representative photomicrographs of HUVEC monolayers incubated for 7 h with CM from 1205Lu cells depleted (siSPARC) or not (siCTRL) for SPARC, compared with control medium. Immunofluorescence for ZO1 (green), F-actin (red) and nuclei (blue) show intercellular gaps between endothelial cells in the presence of siCTRL CM (asterisks). Bar, 20 μm. (g) Quantification of intercellular gaps. Bar graphs show mean±s.e.m (n=7 independent fields).Pvalues shown inb, Unpairedt-test, (c–e,g), two-way analysis of variance. *P<0.05, **P<0.01, ***P<0.001. Figure 1: Tumour-secreted SPARC reduces endothelial monolayer integrity. ( a ) Schematic representation of CM production from melanoma cell cultures. After 24 h, CM was collected and used for permeability assays or mass spectrometry analysis (see Supplementary Fig. 1 and Supplementary Data 1 ). ( b ) Primary endothelial cells (HUVECs) were seeded into gelatin-coated Boyden chambers, allowed to grow to confluence and then treated with TNFα (10 ng ml −1 ) overnight. Permeability was determined by a FITC-Dextran assay 7 h after addition of CM from melanoma cells depleted or not for SPARC by siRNA or from 501Mel cells stably overexpressing SPARC (cl. SPARC) or not (cl. CTRL). Bar graphs show mean±s.e.m., n =2 independent experiments performed in triplicate. Upper panels show representative anti-SPARC blots. Ponceau staining was used as loading control. siCTRL, control siRNA; siSPARC, SPARC siRNA. ( c ) Permeability analysis of human pulmonary microvascular endothelial cells (HPMECs) 7 h after addition of 1205Lu CM depleted or not for SPARC. Bar graphs show mean±s.e.m., n =2 independent experiments performed in triplicate. ( d ) Permeability of HUVECs was assayed using 1205Lu CM cleared from SPARC by immunoprecipitation (IP). Inset shows representative SPARC immunoblot analysis of the cleared CM. Bar graphs show mean±s.e.m., n =2 independent experiments performed in triplicate. ( e ) Permeability assay was performed using CM from 1205Lu cell cultures depleted for SPARC by siRNA and rescued by recombinant human SPARC (rhSPARC). Increasing doses of rhSPARC were added in the upper chamber (2, 5 or 10 μg ml −1 ) and FITC-Dextran fluorescence was determined in the lower chamber 7 h after the addition of CM. Bar graphs show mean±s.e.m., n≥3 independent experiments performed in triplicate. ( f ) Representative photomicrographs of HUVEC monolayers incubated for 7 h with CM from 1205Lu cells depleted (siSPARC) or not (siCTRL) for SPARC, compared with control medium. Immunofluorescence for ZO1 (green), F-actin (red) and nuclei (blue) show intercellular gaps between endothelial cells in the presence of siCTRL CM (asterisks). Bar, 20 μm. ( g ) Quantification of intercellular gaps. Bar graphs show mean±s.e.m ( n =7 independent fields). P values shown in b , Unpaired t -test, ( c – e , g ), two-way analysis of variance. * P <0.05, ** P <0.01, *** P <0.001. Full size image Tumour-derived SPARC induces vascular permeability in vitro To identify the extracellular factors acting on endothelial permeability, we performed a comparative mass spectrometry analysis of serum-free CM prepared from metastatic 1205Lu cells versus non-metastatic 501Mel cells. This analysis revealed that metastatic cells released in the extracellular milieu a pattern of functionally diverse proteins that was qualitatively and quantitatively different as compared with non-metastatic cells ( Supplementary Data 1 ). Notably, several proteins involved in ECM organization (TENA, SPRC, MMP2, TICN1, TIMP2, CSPG2), adhesion (FINC, LAMB1, TSP1/2, ITB1, L1CAM, CD44, ITAV, ITB3), migration and inflammation (IL6, GROA, IL8, TNR1, CCL2) and TGFβ signalling (LTBP3, TGFB1) were dramatically enriched in CM from metastatic 1205Lu cells, whereas proteins associated with a melanocytic profil (PEDF) [17] , K2C8 and K2C18 [18] or skin function (CHLE) [19] , were more abundant in CM from non-metastatic 501Mel cells ( Supplementary Fig. 1b ). Other proteins differentially expressed in 1205Lu CM versus 501Mel included factors involved in additional important tumour cell functionalities such as angiogenesis (NRP1), fibrinolysis (PAI1, GDN, UPAR) or associated with extracellular microvesicles and exosomes (HS90B, RAB7A). The discovery that SPARC, a matricellular protein involved in tumour cell invasion and survival [20] , and endothelial barrier function [21] , was 10-fold more abundant in metastatic melanoma cell CM as compared with CM from a poorly metastatic cell prompted us to investigate whether SPARC contributes to paracrine induction of vascular permeability by melanoma cell-derived CM. We, therefore, engaged different approaches to manipulate SPARC expression and function. First, knockdown of SPARC expression using siRNA strongly attenuated the abilities of CM derived from 1205Lu, A375 and SKMel28 melanoma cell lines or from a short-term culture to promote FITC-Dextran permeability across HUVECs monolayers ( Fig. 1b ). Inhibition of melanoma CM-induced vascular permeability after SPARC knockdown was also evident when FITC-Dextran assays were performed across primary human pulmonary microvascular endothelial cells (HPMECs) monolayers ( Fig. 1c ). Using a complementary approach, we showed that immunodepletion of SPARC protein from melanoma-derived CM impaired its capacity to increase endothelial monolayer permeability ( Fig. 1d ). Conversely, 501Mel cells engineered to overexpress myc-tagged SPARC protein (cl.SPARC) produced CM with higher potential for increasing FITC-Dextran permeability as compared with CM from parental cells ( Fig. 1b ). To test whether the reduced capacity to promote endothelial permeability was a direct consequence of the absence of SPARC in CM, SPARC-silenced CM was rescued by increasing doses of exogenous SPARC. As shown in Fig. 1e , a recombinant tumour source of SPARC was able to rescue dampened endothelial permeability induced by SPARC-silenced CM in a dose-dependent manner. Examination of SPARC secretion by melanoma cells using ELISA (enzyme-linked immunosorbent assay) analyses confirmed that metastatic melanoma cells produced significantly higher levels of SPARC than 501Mel cells or normal melanocytes ( Supplementary Fig. 1c ). Given the emerging role of tumour-derived extracellular vesicles like exosomes in paracrine signalling and endothelial function during metastasis [22] , we verified that SPARC is released as a soluble factor in melanoma culture supernatants of 1205Lu cells. Depletion of exosomal-like particles from culture supernatants by ultracentrifugation indicated that enhanced endothelial permeability function of melanoma CM was maximally mediated by tumour-derived soluble factors. This experiment also demonstrated the non-vesicular origin of SPARC in the CM from 1205Lu cells ( Supplementary Fig. 1d ). Of note, no significant effect of cell density was observed in the regulation of SPARC secretion by 1205Lu melanoma cells ( Supplementary Fig. 2 ). The effect of secreted SPARC on endothelial monolayer integrity was next examined by fluorescence microscopy. HUVECs cells were allowed to grow to form tight monolayers on culture plates. At this point, monolayers were exposed to medium conditioned by 1205Lu cells transfected with control siRNA (siCTRL) or SPARC siRNA (siSPARC). Staining with antibodies against the tight junction component ZO1 or the adherens junction component β-catenin revealed that the monolayer integrity was dramatically perturbed by the addition of CM from control 1205Lu cells ( Fig. 1f and Supplementary Fig. 3a ). Staining of the actin cytoskeleton with phalloidin produced similar observations. In contrast, SPARC-depleted CM displayed severely impaired capacity to disrupt the endothelial barrier and to open intercellular gaps. The formation of intercellular gaps was quantified ( Fig. 1g ) and changes were found significant. When examined on monolayers of lung microvascular cells HPMECs, a similar disrupting activity of SPARC was observed. The opening of intercellular gaps in endothelial monolayers was a direct effect of SPARC as demonstrated by rescue experiments in which exogenous SPARC restored the ability of SPARC-depleted CM to alter endothelial integrity ( Supplementary Fig. 3b,c ). We also examined the functional contribution of SPARC in the induction of vascular permeability in malignant glioma cells, which also rely on its expression for invasive behaviour [23] , [24] . Importantly, SPARC-silenced CM collected from the glioma cell line U87 transfected with SPARC siRNA exhibited disabled potential for increasing endothelial cell permeability ( Supplementary Fig. 4 ). Collectively, these findings support a role for SPARC in tumour cell-induced disruption of endothelial monolayer integrity in vitro . Tumour-derived SPARC alters pulmonary permeability in mice We proceeded further to examine the involvement of SPARC in melanoma cell-induced hyperpermeability of lung capillaries in vivo . Control or SPARC siRNA-treated 1205Lu melanoma cells were injected into nude mice. One day post inoculation, FITC-Dextran was injected into circulation, to measure vessel permeability. After 30 min, the accumulation of the high molecular weight tracer in the lung parenchyma was analysed by fluorescence microscopy ( Fig. 2a,b ). No FITC signal was present in the lungs that were not inoculated with tumour cells. However, FITC-Dextran was detected at significant levels within lungs from mice inoculated with SPARC-competent cells as evidenced by the diffuse areas of fluorescence signal observed in lung sections. In contrast, the intensity of fluorescence was significantly abolished by SPARC silencing ( Fig. 2c ). Permeable Dextran exudation was quantified in the lysates of individual lungs. These analyses confirmed that compared with control cells, vascular permeability was dramatically reduced in lungs from mice inoculated with SPARC-deficient tumour cells, indicating that knockdown of SPARC prevents tumour-induced permeability of lung capillaries ( Fig. 2d ). By contrast, 501Mel cells overexpressing SPARC showed a significant increase in the amount of FITC-Dextran lodged in the lungs compared with parental cells ( Fig. 2e ). These results indicate that SPARC expressed by melanoma cells can disrupt the barrier integrity of lung capillaries. 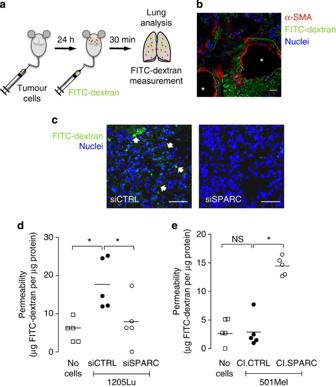Figure 2: Tumour-derived SPARC contributes to lung vascular permeability. (a) Schematic representation of the FITC-Dextran lung extravasation assay procedure. Nude mice were injected into the lateral tail vein with 1205Lu or 501Mel cells modified for SPARC expression. Twenty-four hours post inoculation, mice received 1 mg FITC-Dextran (70 kDa) per 20 g bodyweight intravenously and animals were killed 30 min later. Lungs were perfused free of blood with PBS and fixed for confocal microscopy examination or homogenized for fluorescence measurement. (b) Representative image of lung sections showing extravasated FITC-Dextran (green) after 1205Lu cells inoculation. Sections were stained with antibodies against the vessel wall marker α-SMA (red) and DAPI (blue). Asterisks show microvascular pulmonary lumen. Scale bar, 20 μm. (c) Representative images of lung sections following FITC-Dextran administration in the presence of 1205Lu cells depleted (siSPARC) or not (siCTRL) for SPARC. Sections were stained with DAPI (blue) before confocal microscopy analysis. Arrows show typical accumulation of FITC-Dextran molecules within the lung parenchyma of 1205Lu-injected mice. Scale bar, 100 μm. (d) Quantification of lung microvasculature permeability in the presence of 1205Lu cells depleted (siSPARC) or not (siCTRL) for SPARC. Scatter plots of FITC-Dextran fluorescence in lungs are shown (Dot, single mouse,n=5 mice per group). For each mouse, permeability was reported in micrograms of FITC-Dextran per micrograms of protein from lung homogenates. (e) Quantification of lung microvasculature permeability in the presence of 501Mel cells stably overexpressing SPARC (MelSPARC) or not (MelCTRL) determined as above (n=5 mice per group).Pvalues shown ind, two-way analysis of variance, (e) Kruskal–Wallis test. *P<0.05, **P<0.01. NS, not significant. Figure 2: Tumour-derived SPARC contributes to lung vascular permeability. ( a ) Schematic representation of the FITC-Dextran lung extravasation assay procedure. Nude mice were injected into the lateral tail vein with 1205Lu or 501Mel cells modified for SPARC expression. Twenty-four hours post inoculation, mice received 1 mg FITC-Dextran (70 kDa) per 20 g bodyweight intravenously and animals were killed 30 min later. Lungs were perfused free of blood with PBS and fixed for confocal microscopy examination or homogenized for fluorescence measurement. ( b ) Representative image of lung sections showing extravasated FITC-Dextran (green) after 1205Lu cells inoculation. Sections were stained with antibodies against the vessel wall marker α-SMA (red) and DAPI (blue). Asterisks show microvascular pulmonary lumen. Scale bar, 20 μm. ( c ) Representative images of lung sections following FITC-Dextran administration in the presence of 1205Lu cells depleted (siSPARC) or not (siCTRL) for SPARC. Sections were stained with DAPI (blue) before confocal microscopy analysis. Arrows show typical accumulation of FITC-Dextran molecules within the lung parenchyma of 1205Lu-injected mice. Scale bar, 100 μm. ( d ) Quantification of lung microvasculature permeability in the presence of 1205Lu cells depleted (siSPARC) or not (siCTRL) for SPARC. Scatter plots of FITC-Dextran fluorescence in lungs are shown (Dot, single mouse, n =5 mice per group). For each mouse, permeability was reported in micrograms of FITC-Dextran per micrograms of protein from lung homogenates. ( e ) Quantification of lung microvasculature permeability in the presence of 501Mel cells stably overexpressing SPARC (MelSPARC) or not (MelCTRL) determined as above ( n =5 mice per group). P values shown in d , two-way analysis of variance, ( e ) Kruskal–Wallis test. * P <0.05, ** P <0.01. NS, not significant. Full size image SPARC promotes tumour cell extravasation and lung metastasis Increasing vascular leakiness properties in the lung is an early event in tumour cell extravasation and metastatic colonization. We, therefore, investigated whether the regulation of vascular permeability by tumour SPARC facilitates the passage of melanoma cells across the endothelial barrier and the colonization of lungs by metastatic cells. First, we examined the contribution of SPARC in the interaction of tumour cells with the blood vessel endothelium, a key process for transendothelial migration during extravasation. We attempted to mimic this in vitro by accessing melanoma cell adhesion on a confluent layer of endothelial cells. We found that knockdown or overexpression of SPARC did not significantly affect melanoma cell adhesion to the endothelial monolayer, indicating that melanoma-derived SPARC was dispensable for tumour-endothelial cell adhesion ( Supplementary Fig. 5 ). We then assessed the effects of SPARC knockdown in transendothelial migration of melanoma cell lines (1205Lu and A375) and short-term cultured melanoma cells. When assayed on monolayers of TNFα-activated HUVECs, control siRNA-transfected melanoma cells exhibited ∼ 2- to 3-fold higher rates of migration as compared with their SPARC-silenced counterparts, thereby establishing a strong positive link between SPARC production by melanoma cells and their ability to cross endothelial barriers ( Fig. 3a ). SPARC-silenced 1205Lu melanoma cells also displayed a reduced potential to migrate through monolayers of HPMECs ( Fig. 3b ). The effect of SPARC depletion in cancer cell transmigration was also evidenced in A375 cells stably expressing an inducible SPARC shRNA, and in three other melanoma cell lines ( Supplementary Fig. 6 ) and in U87 glioma cells ( Supplementary Fig. 7 ). In contrast, 501Mel cells overexpressing SPARC exhibited an enhanced capacity to transmigrate across HUVECs monolayers ( Fig. 3c ). Silencing of SPARC in HUVECs monolayers had no significant impact in melanoma transmigration ( Supplementary Fig. 8 ), suggesting that migration of melanoma cell across endothelial monolayers did not require the presence of endothelial-derived SPARC. 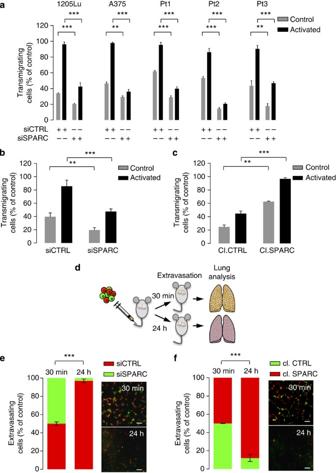Figure 3: Tumour-derived SPARC promotes melanoma cell extravasation. (a) HUVECs grown to confluence on transwell inserts were activated or not (control) with TNFα (10 ng ml−1). CMFDA-stained melanoma cell lines (1205Lu, A375) or short-term cultured melanoma cells (Pt1 to Pt3) transfected with control or SPARC siRNA were seeded onto the inserts. After 7 h, melanoma cell migration across HUVECs monolayers was analysed. Bar graphs show mean±s.e.m. (n=10 random fields from a duplicate determination). Results are representative of at least three independent experiments. (b) Analysis of migration of 1205Lu cells depleted (siSPARC) or not (siCTRL) for SPARC across HPMECs monolayers. Bar graphs show mean±s.e.m. Results are representative of two independent experiments. (c) Analysis of migration of control (cl.CTRL) or SPARC overexpressing (cl.SPARC) 501Mel cells across HUVECs monolayers. Bar graphs show mean±s.e.m. Results are representative of at least three independent experiments. (d) Schematic of the short-term lung colonization assay procedure. Melanoma cells modified or not for SPARC expression were labelled with CMTMR (red) or CMFDA (green) fluorescent dyes. Fluorescent cells were co-injected into tail veins of nude mice, which were killed 30 min or 24 h later. Lungs were collected and at the 24h time point perfused free of blood with PBS to remove intravascular tumour cells. Fluorescently labelled cells in lungs were counted microscopically. (e) Quantification of lung colonization by 1205Lu cells depleted (siSPARC, green) or not (siCTRL, red) for SPARC. The relative proportion of each cell population present within the lungs at the indicated times post injection was determined. Bar graphs show mean±s.e.m. (n=5 randomly chosen fields). Results are representative of two independent experiments. (f) Quantification of lung colonization by control (cl.CTRL, green) or SPARC overexpressing (cl.SPARC, red) 501Mel cells. The relative proportion of each cell population present within the lungs at the indicated times post intravenous injection was determined. Bar graphs show mean±s.e.m. (n=5 randomly chosen fields). Representative images of lungs at 30 min and 24 h are shown. Scale bar, 100 μm.Pvalues shown ina–c, Unpairedt-test, (e,f) Mann–Whitney test. **P<0.01, ***P<0.005. Figure 3: Tumour-derived SPARC promotes melanoma cell extravasation. ( a ) HUVECs grown to confluence on transwell inserts were activated or not (control) with TNFα (10 ng ml −1 ). CMFDA-stained melanoma cell lines (1205Lu, A375) or short-term cultured melanoma cells (Pt1 to Pt3) transfected with control or SPARC siRNA were seeded onto the inserts. After 7 h, melanoma cell migration across HUVECs monolayers was analysed. Bar graphs show mean±s.e.m. ( n =10 random fields from a duplicate determination). Results are representative of at least three independent experiments. ( b ) Analysis of migration of 1205Lu cells depleted (siSPARC) or not (siCTRL) for SPARC across HPMECs monolayers. Bar graphs show mean±s.e.m. Results are representative of two independent experiments. ( c ) Analysis of migration of control (cl.CTRL) or SPARC overexpressing (cl.SPARC) 501Mel cells across HUVECs monolayers. Bar graphs show mean±s.e.m. Results are representative of at least three independent experiments. ( d ) Schematic of the short-term lung colonization assay procedure. Melanoma cells modified or not for SPARC expression were labelled with CMTMR (red) or CMFDA (green) fluorescent dyes. Fluorescent cells were co-injected into tail veins of nude mice, which were killed 30 min or 24 h later. Lungs were collected and at the 24h time point perfused free of blood with PBS to remove intravascular tumour cells. Fluorescently labelled cells in lungs were counted microscopically. ( e ) Quantification of lung colonization by 1205Lu cells depleted (siSPARC, green) or not (siCTRL, red) for SPARC. The relative proportion of each cell population present within the lungs at the indicated times post injection was determined. Bar graphs show mean±s.e.m. ( n =5 randomly chosen fields). Results are representative of two independent experiments. ( f ) Quantification of lung colonization by control (cl.CTRL, green) or SPARC overexpressing (cl.SPARC, red) 501Mel cells. The relative proportion of each cell population present within the lungs at the indicated times post intravenous injection was determined. Bar graphs show mean±s.e.m. ( n =5 randomly chosen fields). Representative images of lungs at 30 min and 24 h are shown. Scale bar, 100 μm. P values shown in a – c , Unpaired t -test, ( e , f ) Mann–Whitney test. ** P <0.01, *** P <0.005. Full size image Using a short-term lung colonization assay to monitor cancer cell extravasation in vivo ( Fig. 3d ), we evaluated whether SPARC levels affect extravasation of tumour cells into lungs. To this end, melanoma cells manipulated to express either low or high levels of SPARC were labelled with two fluorescent dyes, mixed in equal proportions and injected into the tail veins of mice. After 30 min, similar numbers of each co-injected cell population had lodged lungs of the recipient mice. Most SPARC-depleted 1205Lu cells had disappeared from the lungs after 24 h, whereas enforced SPARC expression in 501Mel cells dramatically increased their abilities to extravasate into the pulmonary parenchyma ( Fig. 3e,f ). We next examined the involvement of SPARC in long-term lung colonization using bioluminescent melanoma cells. Control and SPARC siRNA 1205Lu transfectants were injected into the tail veins of mice. Bioluminescence imaging (BLI) immediately post injection confirmed that cells arrested into the lungs. In vivo and ex vivo BLI at the assay end point revealed a dramatic reduction in lung colonization by SPARC knockdown cells compared with control ( Fig. 4a,b ). Quantification revealed an apparent 50-fold reduction in experimental lung metastasis by SPARC knockdown cells. By contrast, overexpression of myc-tagged SPARC in 501Mel cells significantly increased nearly 20-fold lung metastasis ( Fig. 4c ). Immunofluorescence analysis of the expression of myc-tagged SPARC in lung sections showed that individual metastatic lesions retained SPARC expression at the end point of the experiment ( Fig. 4d ). These data suggest that SPARC expression is sufficient to endow 501Mel cells with metastatic competence to lungs. 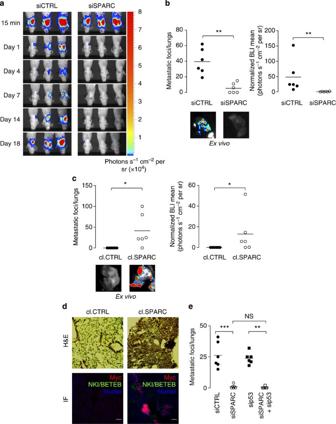Figure 4: Tumour-derived SPARC is required for melanoma lung metastasis. (a) Control and SPARC-depleted 1205Lu LUC+ cells were intravenously injected into nude mice (n=6 mice per group) and lung metastasis was monitored and quantified using a photon imager. Representative images of photon fluxes produced by bioluminescent cancer cells from day 0 to day 18 are shown (three mice per group are shown). Results are representative of three independent experiments. (b)Ex vivoanalysis of lungs from 1205Lu LUC+ siCTRL or siSPARC-injected mice. Scatter plots of lung metastatic foci (left panel, **P=0.0079, Mann–Whitney test) and normalized photon flux (right panel, **P=0.0024, Mann–Whitney test). Dot, single mouse,n=6. Representativeex vivoBLI imaging of lung mets is shown (bottom). (c) Mice were injected with 501Mel LUC+ overexpressing (cl.SPARC) or not (cl.CTRL) myc-tagged SPARC (n=5 mice per group). After 80 days, mice were killed andex vivoanalysis of lungs was performed. Scatter plots of lung metastatic foci (left panel, *P=0.045, Mann–Whitney test) and normalized photon flux (right panel, *P=0.045, Mann–Whitney test). Dot, single mouse,n=5. (d) Histological (haematoxylin and eosin, H&E) and immunofluorescence (IF) analyses of lung sections from mouse injected with 501Mel control or 501Mel overexpressing myc-tagged SPARC after 80 days. Upper panels show a representative H&E staining of lung sections. Lower panels show confocal microscopy images of lung sections labelled with DAPI (blue), antibodies against Myc tag (red) and the melanocytic marker NKI/BETED (green). Scale bar, 500 μm. (e) Depletion of SPARC impairs lung colonization by melanoma cells independently of p53 activation. The 1205Lu LUC+ cells silenced for SPARC (siSPARC), p53 (sip53) or both were injected into nude mice and lung metastasis in each group was monitored until day 18. Scatter plots of lung metastatic foci are shown (**P<0.01, ***P<0.001, two-way analysis of variance. NS, not significant). Dot, single mouse,n=6. Figure 4: Tumour-derived SPARC is required for melanoma lung metastasis. ( a ) Control and SPARC-depleted 1205Lu LUC+ cells were intravenously injected into nude mice ( n =6 mice per group) and lung metastasis was monitored and quantified using a photon imager. Representative images of photon fluxes produced by bioluminescent cancer cells from day 0 to day 18 are shown (three mice per group are shown). Results are representative of three independent experiments. ( b ) Ex vivo analysis of lungs from 1205Lu LUC+ siCTRL or siSPARC-injected mice. Scatter plots of lung metastatic foci (left panel, ** P =0.0079, Mann–Whitney test) and normalized photon flux (right panel, ** P =0.0024, Mann–Whitney test). Dot, single mouse, n =6. Representative ex vivo BLI imaging of lung mets is shown (bottom). ( c ) Mice were injected with 501Mel LUC+ overexpressing (cl.SPARC) or not (cl.CTRL) myc-tagged SPARC ( n =5 mice per group). After 80 days, mice were killed and ex vivo analysis of lungs was performed. Scatter plots of lung metastatic foci (left panel, * P =0.045, Mann–Whitney test) and normalized photon flux (right panel, * P =0.045, Mann–Whitney test). Dot, single mouse, n =5. ( d ) Histological (haematoxylin and eosin, H&E) and immunofluorescence (IF) analyses of lung sections from mouse injected with 501Mel control or 501Mel overexpressing myc-tagged SPARC after 80 days. Upper panels show a representative H&E staining of lung sections. Lower panels show confocal microscopy images of lung sections labelled with DAPI (blue), antibodies against Myc tag (red) and the melanocytic marker NKI/BETED (green). Scale bar, 500 μm. ( e ) Depletion of SPARC impairs lung colonization by melanoma cells independently of p53 activation. The 1205Lu LUC+ cells silenced for SPARC (siSPARC), p53 (sip53) or both were injected into nude mice and lung metastasis in each group was monitored until day 18. Scatter plots of lung metastatic foci are shown (** P <0.01, *** P <0.001, two-way analysis of variance. NS, not significant). Dot, single mouse, n =6. Full size image We recently reported that elevated expression of SPARC favours melanoma survival and growth by inhibiting p53 tumour suppression function [16] . It is, therefore, important to exclude the possibility that the observed decrease in the efficiency of colonization by SPARC-silenced cells was owing to activation of p53-mediated apoptosis. We therefore used p53 siRNA to prevent the death of SPARC-depleted cells. We knocked down p53 along with SPARC in 1205Lu cells and analysed metastatic foci formation 18 days post inoculation into the tail veins of mice. As shown in Fig. 4e , p53 silencing did not significantly affect the dramatic reduction of lung colonization of SPARC-depleted cells. SPARC triggers vascular permeability via endothelial VCAM1 VCAM1 has been identified as an endothelial receptor for leukocyte-derived SPARC [25] . We therefore examined whether the effect of tumour-derived SPARC on disruption of endothelial integrity and extravasation involves VCAM1 signalling. Addition of VCAM1 blocking antibodies to HUVECs monolayers dramatically impaired 1205Lu cell transmigration abilities compared with control antibodies ( Fig. 5a ). Importantly, the presence of VCAM1-blocking antibodies abrogated the enhanced effect of SPARC on transmigration of 501Mel cells. Blockade of VCAM1 also prevented endothelial permeability elicited by melanoma cell CM as assessed by FITC-Dextran method ( Fig. 5b ). We also examined the effect of VCAM-1 knockdown in endothelial cells. Transfection of siRNA targeting VCAM1 resulted in almost complete reduction of VCAM1 protein levels in both resting and TNFα-activated HUVECs ( Fig. 5c ). Knockdown of VCAM1 in activated endothelial cells reduced the opening of intercellular gaps induced by 1205Lu-derived CM and transmigration ( Fig. 5c,d ). Importantly, administration of VCAM1-blocking antibodies before 1205Lu melanoma cells inoculation in mice significantly blocked the development of early lung metastatic colonization ( Fig. 5e ). 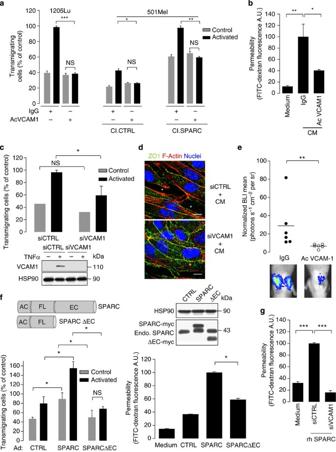Figure 5: Endothelial VCAM1 mediates SPARC-induced vascular permeability and extravasation. (a) Control IgG or VCAM1 blocking antibodies (25 μg ml−1) were added to HUVECs monolayers 1 h before addition of the indicated melanoma cells.In vitrotransendothelial migrations were quantified. Bar graphs show mean±s.e.m.,n=2 independent experiments performed in triplicate. (b) Activated HUVECs monolayers were treated with IgG or VCAM1 blocking antibodies and FITC-Dextran permeability assays were performed using 1205Lu CM. Bar graphs show mean±s.e.m of triplicate determinations. (c) HUVECs transfected with siCTRL or siRNA against VCAM1 were activated or not with TNFα. Transmigration assays were performed with 1205Lu cells. Bar graphs show mean±s.e.m. Results are representative of three independent experiments. Inset shows immunoblot analysis of VCAM1 suppression in HUVECs. (d) Representative confocal microscopy of HUVECs monolayers depleted or not for VCAM1 incubated 7 h with 1205Lu CM. Immunofluorescence for ZO1 (green), F-actin (red) and nuclei (blue) show intercellular gap into the vascular monolayer expressing VCAM1 (asterisks). Bar, 10 μm. (e) Mice were administrated with 25 μg of VCAM1 blocking antibodies or IgG 30 min before inoculation of 1205Lu LUC+ cells. Lung colonization was analyzed after 24 h. Scatter plots of normalized photon flux in lungs. Dot, single mouse,n=6. Representative images of photon fluxes produced by bioluminescent cells are shown. (f) Left, functional domains of SPARC and of the ΔEC mutant. AC, acidic domain; FS, follistatin-like domain and EC, extracellular Ca2+ binding domain. 501Mel cells were infected with control adenovirus (AdCTRL), adenovirus encoding myc-tagged SPARC (AdSPARC) or SPARC mutant deleted of the VCAM1 binding domain (Ad SPARCΔEC). Transendothelial migrations were realized and FITC-Dextran permeability assays were performed using CM from the indicated transduced 501Mel cells. Bar graphs show mean±s.e.m.,n=2 independent experiments performed in triplicate. Expression levels of endogenous SPARC and myc-tagged SPARC transgenes were analysed by immunoblot (right inset). (g) Activated HUVECs monolayers transfected with siCTRL or siVCAM1 were incubated with 5 μg ml−1of rhSPARC for 7 h. Endothelial permeability was assayed using FITC-Dextran. Bar graphs show mean±s.e.m. of triplicate determinations.Pvalues shown ina,candf(left), unpairedt-test, (b,f,(right),g), two-way analysis of variance, (e) Mann–Whitney test. *P<0.05, **P<0.01, ***P<0.005. Figure 5: Endothelial VCAM1 mediates SPARC-induced vascular permeability and extravasation. ( a ) Control IgG or VCAM1 blocking antibodies (25 μg ml −1 ) were added to HUVECs monolayers 1 h before addition of the indicated melanoma cells. In vitro transendothelial migrations were quantified. Bar graphs show mean±s.e.m., n =2 independent experiments performed in triplicate. ( b ) Activated HUVECs monolayers were treated with IgG or VCAM1 blocking antibodies and FITC-Dextran permeability assays were performed using 1205Lu CM. Bar graphs show mean±s.e.m of triplicate determinations. ( c ) HUVECs transfected with siCTRL or siRNA against VCAM1 were activated or not with TNFα. Transmigration assays were performed with 1205Lu cells. Bar graphs show mean±s.e.m. Results are representative of three independent experiments. Inset shows immunoblot analysis of VCAM1 suppression in HUVECs. ( d ) Representative confocal microscopy of HUVECs monolayers depleted or not for VCAM1 incubated 7 h with 1205Lu CM. Immunofluorescence for ZO1 (green), F-actin (red) and nuclei (blue) show intercellular gap into the vascular monolayer expressing VCAM1 (asterisks). Bar, 10 μm. ( e ) Mice were administrated with 25 μg of VCAM1 blocking antibodies or IgG 30 min before inoculation of 1205Lu LUC+ cells. Lung colonization was analyzed after 24 h. Scatter plots of normalized photon flux in lungs. Dot, single mouse, n =6. Representative images of photon fluxes produced by bioluminescent cells are shown. ( f ) Left, functional domains of SPARC and of the ΔEC mutant. AC, acidic domain; FS, follistatin-like domain and EC, extracellular Ca2+ binding domain. 501Mel cells were infected with control adenovirus (AdCTRL), adenovirus encoding myc-tagged SPARC (AdSPARC) or SPARC mutant deleted of the VCAM1 binding domain (Ad SPARCΔEC). Transendothelial migrations were realized and FITC-Dextran permeability assays were performed using CM from the indicated transduced 501Mel cells. Bar graphs show mean±s.e.m., n =2 independent experiments performed in triplicate. Expression levels of endogenous SPARC and myc-tagged SPARC transgenes were analysed by immunoblot (right inset). ( g ) Activated HUVECs monolayers transfected with siCTRL or siVCAM1 were incubated with 5 μg ml −1 of rhSPARC for 7 h. Endothelial permeability was assayed using FITC-Dextran. Bar graphs show mean±s.e.m. of triplicate determinations. P values shown in a , c and f (left), unpaired t -test, ( b , f ,(right), g ), two-way analysis of variance, ( e ) Mann–Whitney test. * P <0.05, ** P <0.01, *** P <0.005. Full size image To further explore the contribution of VCAM1 in tumour-derived SPARC’s effect, we studied the role played by the COOH-terminal extracellular Ca2+ binding (EC) module of SPARC, a domain previously shown implicated in binding to endothelial cells [26] and to VCAM1 (ref. 25 ). 501Mel cells were infected with an adenovirus control or expressing SPARC or SPARC deleted of the EC domain, and transmigration experiments and FITC-Dextran assays were performed. SPARC enhanced transmigration and endothelial permeability capacities of 501Mel cells, whereas the EC domain-deleted mutant was unable to promote these effects ( Fig. 5f ). This strongly suggests that the SPARC EC domain is responsible for mediating endothelial paracrine signalling leading to vascular leakage and tumour cell transmigration. Consistently, ablation of VCAM1 abrogated SPARC-stimulated paracellular permeability, indicating that SPARC likely requires VCAM1 to induce alteration in endothelial barrier integrity ( Fig. 5g ). Leukocyte engagement of VCAM1 on endothelial cells elicits multiple signalling pathways that participate to vascular function including paracellular permeability [27] , [28] . We therefore examined the impact of tumour-derived SPARC on endothelial cell signalling. When HUVECs monolayers were incubated with SPARC-containing CM from 1205Lu cells or A375 cells, activating phosphorylation of SRC, p38 MAPK and myosin light chain 2 (MLC2) were detected in endothelial cells. Compared with resting cells, TNFα-treated HUVECs exhibited augmented levels of p38 and MLC2 phosphorylation ( Fig. 6a and Supplementary Fig. 9a–c ). Importantly, these events were nearly abolished upon incubation of endothelial cells with CM depleted for SPARC by siRNA or immunoprecipitation. Of note, exposure of melanoma CM to endothelial cells did not modulate activation of ERK, JNK, AKT, JAK/STAT or FAK signalling pathways ( Supplementary Fig. 9d and not shown). We next confirmed the p38 MAPK dependence using pharmacological inhibition. In HUVECs treated with the p38 inhibitor SB202190, no phosphorylation of the transcription factor ATF2 and MLC2 was observed following the addition of 1205Lu CM ( Fig. 6b ). Note that SB202190 did not inhibit the 1205Lu CM-induced phosphorylation of the upstream p38 activators, MKK3 and MKK6. The functional relevance of the p38 signalling pathway during SPARC-induced vascular permeability was evidenced by microscopy experiments showing that tumour CM-induced junctional disruption, F-actin increase and paracellular pores formation were prevented by SB202190 ( Fig. 6c ). Finally, inhibition of p38 also impaired transmigration of 1205Lu cells and CM-induced vascular permeability to FITC-Dextran ( Fig. 6d,e ). Together, these experiments demonstrate that interaction of tumour-secreted SPARC with endothelial VCAM1 triggers p38 MAPK signalling towards vascular endothelium permeability and melanoma extravasation. 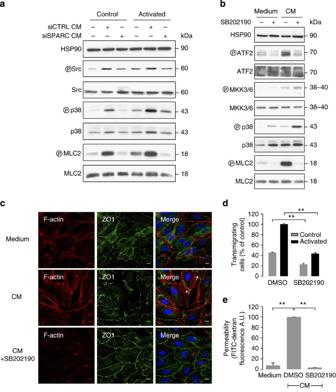Figure 6: SPARC-VCAM1-induced endothelial barrier dysfunction is driven by a p38 MAPK/MLC2 pathway. (a) Immunoblot analysis of HUVECs monolayers activated or not with TNFα and incubated for 7 h with CM from 1205Lu cells depleted or not for SPARC. (b) Immunoblot analysis of HUVECs monolayers untreated or treated with p38 kinase inhibitor SB202190 (10 μM) 1 h before incubation with 1205Lu cell CM compared with medium. (c) HUVECs treated or not with p38 inhibitor SB202190 were incubated with CM from 1205Lu cells or with medium alone. Endothelial monolayers were imaged by confocal microscopy following immunofluorescence staining of ZO1 (green), F-actin (red) and nuclei (blue). Intercellular gaps induced by melanoma CM into the vascular monolayer (asterisks) were absent in SB202190-treated monolayers. Scale bar, 10 μm. (d) Quantification of migration of 1205Lu cells across resting and activated HUVECs monolayers treated or not with p38 inhibitor SB202190 (10 μM) 1 h before addition of melanoma cells. Bar graphs show mean±s.e.m. (n=10 random fields from a triplicate determination). (e) FITC-Dextran permeability assay of HUVECs monolayers untreated or treated with p38 inhibitor SB202190 (10 μM) 1 h before incubation for 7 h with control medium or CM from 1205Lu cells. Bar graphs show mean±s.e.m of triplicate determinations. All the results are representative of at least three independent experiments.Pvalues shown ind, unpairedt-test, (e) two-way analysis of variance. **P<0.01. Figure 6: SPARC-VCAM1-induced endothelial barrier dysfunction is driven by a p38 MAPK/MLC2 pathway. ( a ) Immunoblot analysis of HUVECs monolayers activated or not with TNFα and incubated for 7 h with CM from 1205Lu cells depleted or not for SPARC. ( b ) Immunoblot analysis of HUVECs monolayers untreated or treated with p38 kinase inhibitor SB202190 (10 μM) 1 h before incubation with 1205Lu cell CM compared with medium. ( c ) HUVECs treated or not with p38 inhibitor SB202190 were incubated with CM from 1205Lu cells or with medium alone. Endothelial monolayers were imaged by confocal microscopy following immunofluorescence staining of ZO1 (green), F-actin (red) and nuclei (blue). Intercellular gaps induced by melanoma CM into the vascular monolayer (asterisks) were absent in SB202190-treated monolayers. Scale bar, 10 μm. ( d ) Quantification of migration of 1205Lu cells across resting and activated HUVECs monolayers treated or not with p38 inhibitor SB202190 (10 μM) 1 h before addition of melanoma cells. Bar graphs show mean±s.e.m. ( n =10 random fields from a triplicate determination). ( e ) FITC-Dextran permeability assay of HUVECs monolayers untreated or treated with p38 inhibitor SB202190 (10 μM) 1 h before incubation for 7 h with control medium or CM from 1205Lu cells. Bar graphs show mean±s.e.m of triplicate determinations. All the results are representative of at least three independent experiments. P values shown in d , unpaired t -test, ( e ) two-way analysis of variance. ** P <0.01. Full size image As VCAM1 has been shown to mediate endothelial junction disruption through Rac-dependent production of reactive oxygen species (ROS) and activation of p38 during leukocyte transmigration [29] , ROS levels were monitored in endothelial cells exposed to CM prepared from 1205Lu melanoma cells ( Supplementary Fig. 9e,f ). An increase in ROS production upon exposure of CM was observed compared with control medium. Moreover, we found that pre-incubation with the oxygen scavenger NAC prevented melanoma cell CM-induced activating phosphorylation of p38 and MLC2, providing evidence that p38 activation occurs downstream of ROS. These findings point to a role for ROS as signalling molecules involved in melanoma cell-induced p38 MAPK pathway leading to gap formation and endothelial permeability. SPARC level is associated with human metastatic melanoma Despite earlier studies that have correlated levels of SPARC to the early stages of malignant melanomas and found expression of SPARC associated with invasion and poor clinical income [30] , [31] , [32] , no evidence has been provided for an association of SPARC with distant melanoma metastases. To determine the clinical relevance of our findings, we investigated SPARC expression in human melanoma lung metastases and amounts of circulating SPARC in blood from patients with stage 4 metastatic disease. SPARC level in lung metastasis samples from patients with metastatic melanoma (MM) was analysed by IHC. In four of four samples evaluated, a strong SPARC immunoreactivity was detected in association with metastatic melanoma cells. Strikingly, no expression of SPARC was found in non-tumoral stroma of lung tissues ( Fig. 7a ). Regarding the high expression of SPARC found in melanoma lung metastases, we thus sought evidence for a potential link between SPARC expression and advanced melanoma. We measured the SPARC level in serum from nine MM patients and eight healthy volunteers, and found a statistically significant increase of SPARC in clinical samples (1.01±0.28 μg ml −1 ) versus control individuals (0.67±0.17 μg ml −1 ) ( Fig. 7b ). Human SPARC circulating levels were also detected in melanoma-xenografted mice bearing lung metastases in comparison with tumour-free mice ( Supplementary Fig. 10 ). Results with clinical samples are in agreement with our functional observations pointing to a critical role of SPARC during paracrine remodelling of the vascular endothelium by circulating cancer cells. In addition, our results identified VCAM1 as a central ligand for tumour-derived SPARC during malignant endothelium disruption and melanoma cell extravasation in lungs. Our mechanistic findings are summarized in the schematic Fig. 7c . 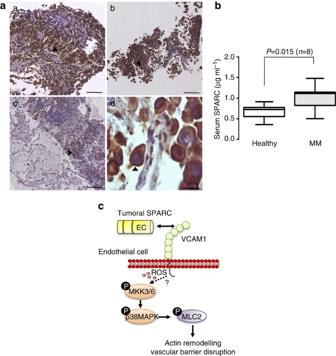Figure 7: SPARC is associated with distant metastasis in human melanoma. (a) Immunohistochemical staining for SPARC in lung melanoma metastases from patients (n=4). Photomicrographs of melanoma metastases at low-power magnification (a–c) and high-power magnification (d). Arrowheads point to SPARC positive tumour cells whereas asterisks show SPARC negative non-tumoral tissues. Scale bars, 100 μm (a), 200 μm (b and c) , 2 μm (d). (b) Serum analysis for SPARC from metastatic melanoma (MM) patients compared with healthy donors (n=8;P=0.015, Mann–Whitney test). Error bars represent mean±s.e.m (c) Schematic model depicting how tumour-derived SPARC triggers endothelial permeability. SPARC binding to VCAM1 promotes actin remodelling and opening of endothelial junctions through a ROS-MKK3/6-p38MAPK-MLC2 signalling pathway. Figure 7: SPARC is associated with distant metastasis in human melanoma. ( a ) Immunohistochemical staining for SPARC in lung melanoma metastases from patients ( n =4). Photomicrographs of melanoma metastases at low-power magnification (a–c) and high-power magnification (d). Arrowheads point to SPARC positive tumour cells whereas asterisks show SPARC negative non-tumoral tissues. Scale bars, 100 μm (a), 200 μm (b and c) , 2 μm (d). ( b ) Serum analysis for SPARC from metastatic melanoma (MM) patients compared with healthy donors ( n =8; P =0.015, Mann–Whitney test). Error bars represent mean±s.e.m ( c ) Schematic model depicting how tumour-derived SPARC triggers endothelial permeability. SPARC binding to VCAM1 promotes actin remodelling and opening of endothelial junctions through a ROS-MKK3/6-p38MAPK-MLC2 signalling pathway. Full size image Metastasis arises via a complex succession of events, which involves dissemination and growth of cancer cells to distant organs. Many of these complex events are orchestrated by molecular pathways operating within the malignant cells, and by interactions between tumour cells and non-neoplastic stromal cells. The ability of a circulating tumour cell to escape the vasculature and extravasate into the parenchyma of distant sites is one of the rate-limiting steps of the metastatic cascade [33] . This step requires dynamic tumour–endothelium communication through the release of vascular permeability factors to breach the endothelial barrier, thereby enabling the passage of the tumour cell across the endothelium. The identification of such tumour-derived permeability factors will provide new mechanistic insights into metastasis, thereby offering new therapeutic opportunities. To address these challenges, we assumed that highly metastatic melanoma cells release in their extracellular milieu a spectrum of proteins that should differ quantitatively and/or qualitatively from poorly metastatic cells. We thus used mass spectrometry to identify novel extracellular tumour factors acting on endothelial permeability. Our approach revealed in CM from metastatic melanoma the presence of biological factors, such as CCL2 (ref. 34 ), TGF-β [35] , IL8 (ref. 36 ) and matrix metalloproteinases [37] , which were previously implicated in tumour-mediated disruption of endothelium integrity. Notably, angiopoietin-like 4, a matricellular protein endowing breast tumours with the capacity to disrupt lung capillaries and seed pulmonary metastases [35] , [38] , was absent from our proteomic analysis. In line with this, angiopoietin-like 4 was reported to prevent metastasis of melanoma B16 cells by inhibiting vascular permeability and tumour cell motility [39] . One other matricellular protein emerging from our differential screen is SPARC. A previous proteomic analysis identified high levels of SPARC associated with metastatic melanoma secretomes [40] . Our comparative proteomic analysis corroborates this report, but further extends the notion that SPARC is associated with melanoma progression by showing differential levels of secreted SPARC between untransformed melanocytes, poorly metastatic and highly metastatic melanoma cells ( Supplementary Fig. 1 ). Early studies have shown a role for SPARC in vascular biology in non-malignant settings [21] , [41] . However, its importance in the regulation of tumour-initiated vascular endothelial permeability has remained poorly studied. Therefore, we tested the possibility that melanoma-derived SPARC represents a novel permeability factor favouring tumour cell extravasation during haematogenous metastasis. We showed that expression of SPARC is sufficient to endow melanoma cells with the ability to disrupt the integrity of lung capillaries and extravasate into the pulmonary parenchyma, which has not been reported before. Strikingly, our results indicate that metastatic melanoma cells exert their pathological inhibitory effects on endothelial integrity in large part through SPARC secretion. Indeed, in the absence of tumour SPARC, no significant compensatory mechanisms were observed in our different experimental settings modelling in vitro and in vivo endothelial permeability and melanoma cell extravasation during lung metastatic dissemination. SPARC (also known as osteonectin) is a multifunctional adaptor protein operating both in physiological processes such as development and tissue remodelling, and pathological conditions like cancer. SPARC regulates cell–cell and cell–matrix interactions in cell type- and context-dependent manner. In the tumour microenvironment, both neoplastic and neighbouring stromal cells can produce SPARC, thereby imparting a complexity of action for SPARC in cancer. In melanoma, we and others have previously identified an autocrine role for SPARC in regulating invasiveness, epithelial-mesenchymal-like transition and melanoma survival [14] , [15] , [16] , [42] . Although SPARC expression has been clearly linked to cancer progression through cell-autonomous and non-autonomous actions in cell invasion and survival [20] , [43] , [44] , its function as a paracrine factor has remained poorly characterized. Paracrine functions attributed so far to SPARC in melanoma were related to inhibition of polymorphonuclear leukocyte recruitment [43] , and inhibition of proliferation and migration capacities of endothelial cells in vitro [45] . Supported by previous evidence that elevated SPARC is associated with the occurrence of distant metastases and poor survival in melanoma patients [30] , [31] , our findings functionally demonstrate that SPARC mediates critical tumour cell–endothelium communications through a novel paracrine function on lung capillaries culminating in breaching vascular integrity during metastatic dissemination. Clinically, our findings are underlined by the high expression of SPARC that we observed in pulmonary metastases of melanoma biopsies. Interestingly, a recent study found SPARC overexpressed mainly in lung metastases from melanoma as compared with other primary tumours [46] . Although endothelial cells in the tumour microenvironment are known to produce high levels of SPARC, we found that endothelial-derived SPARC did not influence melanoma cell transmigration, further supporting the notion that tumour- and host-derived SPARC have different biological activities and that the origin of SPARC participates to the complexity of SPARC in metastasis [44] , [47] . The question remains whether secreted SPARC has the ability to exert a similar task on endothelial permeability in other virulent cancers. Our findings indicate that this is indeed the case for malignant glioma, a tumour that, like melanoma, has a neuroectodermal origin. Also, the observation that SPARC belongs to a gene signature bestowing lung metastasis virulence to breast cancer [48] further adds to the paracrine influence of tumour SPARC in the metastatic disease. However, in contrast to breast cancer in which SPARC has no role in primary tumour growth, in melanoma, SPARC provides survival advantages in the primary tumour [14] , [16] as well as metastatic competence. Recruitment of various circulating blood cells such as macrophages, neutrophils or platelets by tumour-derived factors has been recognized to assist tumour cell extravasation at metastatic sites [8] , [49] . In this regard, CCL2 that we identified in our proteomic analysis, was recently shown to attract myeloid-derived monocytes and to promote efficient colon cancer cell extravasation [34] . Whether metastasizing melanoma cells rely on SPARC for cooperative interactions with circulating blood cells enabling efficient extravasation across the vascular barrier remains to be determined. Mechanistically, we demonstrate that SPARC activates VCAM1 on endothelial cells, thereby disrupting intercellular junctions to enable the transmigration of melanoma cells and efficient extravasation into the lung parenchyma. VCAM1 is a transmembrane endothelial glycoprotein, which plays a critical role during inflammatory reaction by permitting the recruitment of leukocytes at the inflammatory sites. It contributes to the rolling and adhesion of leukocytes during the process of leukocyte diapedesis via high-affinity binding to its counter receptor α4ß1 expressed at the leukocyte cell surface [27] , [28] . Another contributor to VCAM1-mediated leukocyte diapedesis was identified as being SPARC [25] . In addition, our data establish that SPARC contributes to the function of VCAM1 during melanoma cell extravasation. Importantly, neither knockdown nor overexpression of SPARC affected the adhesion of melanoma cells in vitro , indicating that SPARC is dispensable for tumour cell adhesion to the endothelial monolayer, a process relying on α4ß1/VCAM1 interaction [50] . Instead, we show that interaction between SPARC and VCAM1 activates signalling pathways driving endothelial paracellular permeability, a key process facilitating tumour cell diapedesis. Our present results reveal an unprecedented role for paracrine stimulation of endothelial cells by tumour-secreted SPARC and the contribution of VCAM1 in this process. The signalling processes that control opening of the endothelial barrier and vascular integrity are highly complex. Physiological and pathological pathways that increase endothelial permeability act through disruption of intercellular junctions and acto–myosin contractibility [8] . A survey of signalling pathways activated by SPARC-competent melanoma CM on endothelial cells identified the p38 MAPK pathway as responsible for tumour-induced actin cytoskeleton remodelling and intercellular pores formation. Activation of p38 MAPK signalling route in endothelial cells by extravasating tumour cells has been observed previously in colon carcinoma cells [34] . In our study, SPARC-mediated VCAM1 activation was found to stimulate SRC tyrosine kinase activity and p38-dependent MLC2 phosphorylation. The effect of SPARC-competent melanoma CM on SRC activation is consistent with an earlier study showing that purified SPARC affects endothelial junction through a tyrosine phosphorylation-dependent signalling pathway [51] . Phosphorylation of MLC2 leads to increased acto–myosin crossbridging, force development and subsequent contraction in endothelial cells. The ensuing cell retraction promotes gap formation and vascular permeability [52] . Previous studies have shown that antibody-mediated crosslinking of VCAM1 stimulated a Rac/ROS/p38 signalling cascade in endothelial cell during leukocyte transmigration [29] . Accordingly, we found that intracellular ROS production contributes to activation of p38 MAPK and MLC2 in endothelial cells stimulated by SPARC-competent melanoma secretome. We can thus propose that activation of VCAM1 by tumour-derived SPARC uses a similar molecular route to open endothelial barrier and facilitates melanoma cell transmigration. In addition, the disruption of adherens junctions following VE-cadherin disassembly has also been reported to rely on p38 MAPK signalling pathway [53] , pointing to the central role of this pathway in tumour-induced vascular permeability. In conclusion, we discovered a new mechanism by which circulating melanoma cells can escape vasculature locations to establish metastases. Our findings demonstrate that SPARC functions through endothelial VCAM1 as a major tumour permeability factor produced by metastatic melanoma cells. SPARC has the ability to disrupt the integrity of vascular endothelial cell layers both in vitro and in the lungs, facilitating the passage of melanoma cells and their colonization. Importantly, our data offer a biochemical explanation for the long-known clinical association of SPARC expression with distant metastasis and poor outcome in melanoma patients. Tumour-secreted SPARC thus emerges as a multifunctional mediator of metastatic development contributing to tumour cell dissemination at the primary site and extravasation at distant sites. Our study provides a rationale and mechanistic basis for targeting SPARC–VCAM1 interaction and their downstream target p38 MAPK to treat the metastatic disease. Cells and reagents Human A375, 1205Lu and SKMel28 melanoma cell lines were obtained from ATCC. Human 501Mel cells, kindly supplied by Ruth Halaban were described elsewhere [42] . Human WM9 and WM793 cell lines were the kind gift of Meenhard Herlyn and have been previously described [42] . Patient melanoma cells (Pt1, Pt2 and Pt3) were the kind gift of Robert Ballotti and prepared as previously described [54] . Melanoma cells were cultured in Dulbecco’s modified Eagle Medium (DMEM) plus 7% FBS (HyClone). Human U87 glioma cells, generously provided by Dominique Figarella-Branger and Ellen Van Obberghen-Schilling were maintained in DMEM supplemented with 7% FBS. Human primary epidermal melanocytes are from our lab stock and maintained as described previously [15] . The 501Mel cells expressing a myc-tagged SPARC (501Mel cl.SPARC) or carrying an empty expression cassette of pcDNA3 vector (501Mel cl.CTRL) have been described [16] . For in vivo bioluminescence imaging, 1205Lu LUC+, 501Mel cl.CTRL LUC+ and 501Mel cl.SPARC LUC+ cells were obtained by lentiviral transduction (pLenti6/V5-D-TOPO; Life Technologies) and blasticidin selection (2 μg ml −1 ). HUVECs and HPMECs were obtained from Lonza and PromoCell, respectively. Endothelial cells were cultured in complete EGM2 BulletKit medium supplemented with 2% FBS (HUVECs) or 5% FBS (HPMECs) and full supplements (Lonza) and were used between —two to six passages. Culture reagents were purchased from Life Technologies. The selective inhibitor of p38 MAP kinase SB202190 was from Tocris Bioscience. An equal amount of DMSO was used as vehicle control. CellTracker CMFDA and CMTMR dyes (Molecular Probes), and FITC-Dextran (70,000 MW) were purchased from Life Technologies. Recombinant human SPARC purified from mouse myeloma cells was purchased from R&D System. All other reagents were obtained from Sigma-Aldrich unless stated otherwise. Preparation of conditioned medium Melanoma cells were grown to ∼ 80% confluence in growth culture medium. Following washes in EGM2 medium (Lonza), cells were incubated for 24 h in defined endothelial cell medium EGM2 with full supplements and 2% FBS (BulletKit, Lonza) at 37 °C. Medium conditioned by melanoma cells was then harvested, centrifuged at 2,500 g for 5 min and filtrated by 0.22-μm filters to eliminate cell debris. The preparation of CM for mass spectrometry analysis is described in Supplementary Methods . In some experiments, extracellular vesicle-depleted culture supernatants were prepared by differential ultracentrifugation as described [55] . To specifically deplete SPARC from melanoma CM, we performed immunoprecipitation experiments. Briefly, CM from 1205Lu cells was incubated overnight with 15 μg of polyclonal anti-hSPARC antibody (R&D System) or control IgG (Dako) pre-absorbed to protein G-agarose at 4 °C. The cleared CM was collected and added to endothelial cell monolayer for in vitro permeability assays. In vitro vascular permeability assay A total 1 × 10 5 HUVECs or HPMECs were seeded onto gelatin-coated Transwell inserts (8 μm pore size, Corning), and allowed to grow in complete EGM-2 endothelial medium to confluence for 4 days. Endothelial cell monolayers were subsequently stimulated for 16 h with TNFα (10 ng ml −1 ; PeproTech). CM from various melanoma cells or EGM2 medium alone (EGM2 BulletKit, 2% FBS) mixed with FITC-Dextran 70,000 MW (0.05 mg ml −1 ) was then added to the upper chamber of the Transwell. Permeability was monitored by the endothelial transcellular passage of FITC-Dextran 7 h later on a Fluoroskan microplate reader. For neutralizing VCAM1 antibody experiments, TNFα-activated endothelial cell monolayer were pre-treated for 1 h with anti-human VCAM1 blocking antibody (R&D System) or IgG isotype control (25 μg ml −1 each). RNAi studies and viral transductions Negative control, SPARC, VCAM1 and p53 Stealth RNAi siRNA duplexes were designed by Invitrogen (Life Technologies). Please see Supplementary Table 1 for the corresponding siRNA sequences. Transfection of siRNA was carried out using Lipofectamine RNAiMAX (Life Technologies), at a final concentration of 50 nM. Unless stated otherwise, cells were assayed 3 days post transfection. A375 cells stably expressing doxycycline-inducible SPARC short hairpin RNA (shRNA) were described previously [16] . Adenoviruses carrying an empty expression cassette of pcDNA3 vector, used as control (AdCTRL) or expressing SPARC (AdSPARC) or a SPARC truncation mutant (SPARCΔEC) with a myc-tag at their carboxyl terminus have also been described previously [15] . Immunoblot analysis and antibodies Melanoma cells were collected as described before [16] . Endothelial cells were lysed in RIPA buffer (50 mM Tris-HCl (pH 7.4); 150 mM NaCl; 1% NP40; 0.1% SDS; 0.5% deoxycholate) supplemented with protease inhibitors and phosphatase inhibitors (Roche Diagnostics) and briefly sonicated. Whole-cell lysates were subjected to SDS–PAGE and immunoblot analysis. The following antibodies were used at working dilution of 1:1,000, unless otherwise mentioned: anti-SPARC (Haematologic Technologies), anti-HSP90 (Santa Cruz Biotechnology), anti-VCAM1 (Santa Cruz Biotechnology, dilution 1:200), anti-Fibronectin (Sigma), anti-VE-cadherin (Zymed, dilution 1:250), anti-p38, anti-phospho-p38 (Thr180/Tyr182), anti-MLC2, anti-phospho-MLC2 (Ser19) (dilution 1:500), anti-ATF2 (dilution 1:500), anti-phospho-ATF2 (Thr69/71) (dilution 1:500), anti-MKK3/6, anti-phosho-MKK3 (Ser189)/MKK6 (Ser207), anti-SRC, anti-phospho-SRC (Tyr416), anti-FAK, anti-phospho-FAK (Tyr397), anti-phospho-AKT (Ser473), anti-phospho-SAPK/JNK (Thr183/Tyr185) and anti-phospho-ERK1/2 (Thr202/Tyr204) were from Cell Signaling Technology. Peroxidase-conjugated anti-mouse and anti-rabbit antibodies were from Cell Signaling Technology. Peroxidase-conjugated anti-goat antibody was from Dako. Secondary antibodies were used at 1:3,000 dilution. Proteins were detected by enhanced chemiluminescence (ECL) Amersham Western Blotting Detection Reagents (GE Healthcare Life Sciences). Original images of blots are provided in Supplementary Figs 11–13 . Fluorescence and confocal microscopy Endothelial cells were grown to confluence on gelatin-coated glass coverslips. After the indicated treatments, cell monolayers were rinsed briefly in phosphate-buffered saline (PBS), fixed in 4% formaldehyde for 15 min, and incubated with primary antibodies against Z01 (1:100; Zymed) or β-catenin (1:100; BD Biosciences) overnight at 4 °C in humidified chambers in a solution containing 0.2% saponin and 1% BSA. Cells were washed, incubated with Alexa Fluor-conjugated secondary antibodies (1:1,000; Molecular Probes) and mounted in ProLong Gold Antifade Reagent with DAPI (Life Technologies). For actin staining, fixed cells were incubated with Texas Red-X phalloidin (1:100; Molecular Probes) for 1 h at room temperature. Images were captured on a Zeiss LSM 510 META laser-scanning confocal microscope, with sequential fluorophore excitation. In vivo experiments All mouse experiments were carried out in accordance with the Institutional Animal Care and the local ethics committee (CIEPAL-Azur agreement NCE/2014-179). Lung microvasculature permeability was determined by the FITC-Dextran extravasation technique as previously described [35] . Briefly, 5-week-old female athymic (nu/nu) mice (Harlan) were intravenously injected with 1205Lu cells (1 × 10 6 ) resuspended in 100 μl of PBS. Twenty-four hours post inoculation, mice were intravneously injected with FITC-Dextran 70,000 MW at 1 mg per 20 g body weight, followed by euthanasia 30 min later. Lungs were perfused with PBS, dissected and homogenized for fluorescence quantification of the tracer or fixed in 4% paraformaldehyde and frozen. Cryosections of lungs (8 μm) were stained with an antibody against the vessel wall marker α-SMA (1:100; Abcam) and examined by fluorescence microscopy for FITC-Dextran extravasation. Images were acquired on a Zeiss LSM 510 META laser-scanning confocal microscope. Lung homogenates were prepared in RIPA buffer supplemented with protease inhibitors and phosphatase inhibitors, briefly sonicated and quantified using a protein assay kit (Bio-Rad) according to the manufacturer’s manual. Fluorescence was measured in lung homogenates using a Fluoroskan microplate reader (excitation, 485 nm; emission, 530 nm). Quantification of extravasated FITC-Dextran was determined in lung homogenates from different animals and calculated against a FITC-Dextran standard curve. Data are expressed as μg of FITC-Dextran per μg of protein from lung homogenates. For short-term lung colonization assays, melanoma cell populations were differentially labelled with 5 μM CellTracker Green CMFDA or CellTracker Orange CMTMR dyes as described [56] . Equal numbers (7.5 × 10 5 ) were co-injected into the tail veins of nude mice, which were killed 30 min or 24 h later. At 24 h, lungs were flushed and perfused free of blood with PBS to remove intravascular tumour cells. Fluorescently labelled cells in lungs were counted microscopically. For experimental lung metastasis studies, 1 × 10 6 melanoma cells engineered to express a luciferase reporter gene (LUC+ cells) were resuspended in 100 μl of PBS and injected into the tail veins of nude mice. Lung metastasis was monitored and quantified using BLI. Mice were anesthetized and injected intraperitoneally with 50 mg kg −1 D-luciferin (PerkinElmer) in PBS. Images were acquired using a Photon Imager (Biospace Lab) system and data analysed with the M3Vision software (Biospace Lab). The total numbers of photons per second per steradian per square centimeter were recorded. For BLI plots, photon flux was calculated for each mouse by using a rectangular region of interest encompassing the thorax of the mouse in a prone position. This value was normalized to the value obtained immediately after injection (15 min), so that all mice had an arbitrary starting BLI signal of 100. Mice were imaged twice a week. For ex vivo BLI, lungs harvested and perfused with PBS were immersed in D-luciferin diluted in PBS to a final concentration of 5 mg ml −1 for 5 min before imaging. For immunostaining of metastases, lungs were perfused with PBS, fixed in 4% paraformaldehyde, OCT-embedded (Gentaur) and cryosectioned. Sections of lungs (8 μm) were stained with haematoxylin and eosin or incubated with antibodies against myc (1:100; Cell Signaling Technologies) and NKI/BETEB (1:20; Hycult Biotech) before detection with Alexa Fluor-conjugated secondary antibodies (1:1,000; Molecular Probes). Sections were mounted in ProLong Gold Antifade Reagent with DAPI (Life Technologies). Images were acquired on a Zeiss (PALM) microscope. In the study with VCAM1-blocking antibody, 25 μg of anti-mouse VCAM1 antibody (eBioscience) or IgG isotype control were administrated through tail vein injection 30 min before 1205Lu LUC+ inoculation. Lung extravasation at 24 h was monitored and quantified by bioluminescence imaging, as described above. Transendothelial migration A total 1 × 10 5 HUVECs or HPMECs were plated in the upper chamber of a gelatin-coated Transwell insert and grown in complete endothelial medium to confluence. The endothelial monolayer was then left untreated or treated with human TNFα (10 ng ml −1 ) for 16 h. Melanoma cells were pulsed with 5 μM CellTracker Green CMFDA dye for 30 min, detached by HyQTase treatment (HyClone) and plated on top of the endothelial monolayer. Cells were allowed to migrate for 7–24 h at 37 °C in 5% CO 2 . Complete EGM2 medium plus 10% FBS was used as a chemoattractant. The Transwells were then fixed in 4% paraformaldehyde, cells on the apical side of each insert were scraped off, and the Transwell membrane mounted onto glass slides. Migration to the basolateral side of the membrane was visualized with a Zeiss (PALM) immunofluorescent microscope at × 5 magnification. Pictures of five random fields were captured for quantification using NIH ImageJ analysis software. All the experiments were performed in duplicates and repeated at least three times. Tumour-endothelial cell adhesion assay The adhesion assays were performed in black 96-well culture dishes in triplicate. HUVECs were seeded onto gelatin, allowed to grow to confluence for 4 days and stimulated for 16 h with TNFα (10 ng ml −1 ). Melanoma cells were pulsed with 5 μM CellTracker Green CMFDA for 30 min and collected by HyQTase treatment. Fluorescent dye-labelled cells were then allowed to adhere onto the endothelial cell monolayer for 7 h. Non-adherent cells were removed by washing with PBS supplemented with 1 mM CaCl 2 and 1 mM MgCl 2 and fluorescence was measured. Data are expressed as the percentage of adherent cells per total cells. Detection of ROS by flow cytometry ROS levels were measured using the redox-sensitive dye CM-H 2 DCFDA (Molecular Probes, Life Technologies). The green fluorescence was collected using a Miltenyi Biotec flow cytometer and the MACSQuantify software for acquisition and analysis. Human samples and immunohistochemistry Lung metastatic melanoma specimens were obtained from Histopathology and Dermatology Departments of Nice University Hospital. Informed written consent was obtained from all the patients in accordance with the Declaration of Helsinki to the use of human biological samples for research purposes. Formalin-fixed, paraffin-embedded tissue blocks were retrieved from the archive and analysed by IHC. The SPARC polyclonal antibody (1:100; R&D System) was incubated with tissue sections (2 μm) after heat-induced epitope retrieval (pH 6.0). The samples were incubated with primary antibody, followed by incubation with a secondary antibody conjugated to peroxidase (1:100; Dako). Detection was performed using diaminobenzidine for 8 min, and the slides were counterstained with haematoxylin. ELISA assay The concentration of SPARC in various CM of melanoma cell lines or serum samples were quantified using the human SPARC Quantikine ELISA kit (R&D Systems) as per the manufacturer’s protocol. After receiving their informed consent, we obtained sera from nine patients with metastatic melanoma treated at the Department of Dermatology, Nice University Hospital, France. Eight healthy volunteers were recruited as controls. Results from two independent experiments were normalized. Statistics Unless otherwise stated, all the experiments were repeated at least three times and representative data/images are shown. Statistical data analysis was performed using GraphPad Prism 5 software. Unpaired two-tailed Student’s t -test and Mann–Whitney test were used for statistical comparisons between the two groups and Kruskal–Wallis test with Dunn post tests or two-way analysis of variance test with Bonferroni post tests to compare three or more groups. Error bars are±s.e.m. How to cite this article: Tichet, M. et al. Tumour-derived SPARC drives vascular permeability and extravasation through endothelial VCAM1 signalling to promote metastasis. Nat. Commun. 6:6993 doi: 10.1038/ncomms7993 (2015).